Switch of PKA substrates from Cubitus interruptus to Smoothened in the Hedgehog signalosome complex Hedgehog (Hh) signalling is crucial for developmental patterning and tissue homeostasis. In Drosophila , Hh signalling is mediated by a bifunctional transcriptional mediator, called Cubitus interruptus (Ci). Protein Kinase A (PKA)-dependent phosphorylation of the serpentine protein Smoothened (Smo) leads to Ci activation, whereas PKA-dependent phosphorylation of Ci leads to the formation of Ci repressor form. The mechanism that switches PKA from an activator to a repressor is not known. Here we show that Hh signalling activation causes PKA to switch its substrates from Ci to Smo within the Hh signalling complex (HSC). In particular, Hh signalling increases the level of Smo, which then outcompetes Ci for association with PKA and causes a switch in PKA substrate recognition. We propose a new model in which the PKA is constitutively present and active within the HSC, and in which the relative levels of Ci and Smo within the HSC determine differential activation and cellular response to Hh signalling. In many developmental processes, Hh induces differential cell fates as a function of its concentration [1] . During Drosophila wing development, for example, posterior compartment (P) cells secrete Hh, which then establishes a local activity gradient in the anterior compartment (A) cells and leads to the formation of several different cell types ( Fig. 1d ). 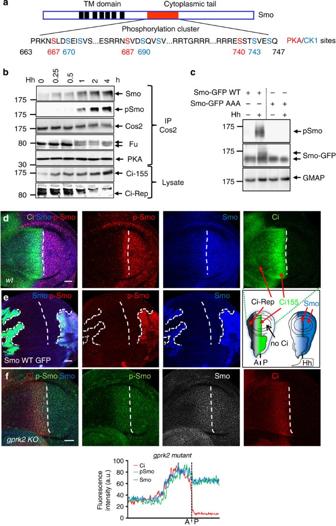Figure 1:In vitroandin vivodetection of a PKA-dependent phospho-Smo isoform. (a) Schematic representation of the Smo protein. (b) Endogenous Cos2 immunoprecipitation and western blot analysis showing a kinetic of Hh signalling in cl8 cells at different time point. (c) Smo-GFP WT or Smo-GFP AAA were immunoprecipitated from S2R+ cells, and analysed for the presence of p-Smo, Smo and GMAP (control). (d–f) Wing imaginal discs were stained for Ci (green,d, and red,f,), p-Smo (red,d,eand green,f) and Smo (blue,d–fand grey,f). Ind, scheme of Hh pathway in wing imaginal discs. (e) Wing discs expressing UAS Smo WT clones (marked by the presence of GFP). (f)gprk2 KOwing discs. Note that in the anterior cells activated by Hh, there is a gradient of Smo, pSmo patterns and Ci155 stabilization with a similar slope, as shown on the graphf. In each of the figures, wing discs are shown with ventral on the top and posterior on the right; the A/P and D/V borders are indicated by dashed lines. Scale bars, 20 μm. Figure 1: In vitro and in vivo detection of a PKA-dependent phospho-Smo isoform. ( a ) Schematic representation of the Smo protein. ( b ) Endogenous Cos2 immunoprecipitation and western blot analysis showing a kinetic of Hh signalling in cl8 cells at different time point. ( c ) Smo-GFP WT or Smo-GFP AAA were immunoprecipitated from S2R+ cells, and analysed for the presence of p-Smo, Smo and GMAP (control). ( d – f ) Wing imaginal discs were stained for Ci (green, d , and red, f ,), p-Smo (red, d , e and green, f ) and Smo (blue, d – f and grey, f ). In d , scheme of Hh pathway in wing imaginal discs. ( e ) Wing discs expressing UAS Smo WT clones (marked by the presence of GFP). ( f ) gprk2 KO wing discs. Note that in the anterior cells activated by Hh, there is a gradient of Smo, pSmo patterns and Ci155 stabilization with a similar slope, as shown on the graph f . In each of the figures, wing discs are shown with ventral on the top and posterior on the right; the A/P and D/V borders are indicated by dashed lines. Scale bars, 20 μm. Full size image Several integral membrane proteins are involved in Hh signal reception, including Patched (Ptc) [2] , [3] , which binds to Hh, and Smoothened (Smo), a G protein-coupled receptor that transduces the signal [4] . In Drosophila , the binding of Hh with its receptor Ptc causes increase of Smo level and plasma membrane localization [5] , [6] , where it recruits the Hh signalling complex (HSC) [7] , [8] , [9] , [10] composed of the protein kinase A (PKA) [11] , the kinesin-like protein Costal2 (Cos2) [12] , [13] , the serine/threonine kinase Fused (Fu) [14] and the zinc-finger transcription factor Cubitus interruptus (Ci; Gli in vertebrates) [15] , [16] . Hh signalling is mediated by the Ci/Gli activity with the levels of Hh signalling being proportional to the ratio of the activator form of Ci (CiA or GliA) to the repressor form (Ci-Rep or GliR) [1] . During the activation of the pathway, Smo undergoes phosphorylations, which occur mainly at its carboxy-terminal cytoplasmic tail (C-tail) [17] , [18] , [19] . These modifications are necessary for the dimerization of the two C-tails within the Smo homodimer, which promotes the activation of Hh signalling [20] , [21] . Moreover, phosphorylations are also required to regulate Smo cell-surface accumulation in response to Hh [18] . The kinases involved in this process are the PKA, the casein kinase 1 (CK1), the casein kinase 2 (CK2) and the GPR kinase 2 (GPRK2) [22] , [23] with PKA acting as a primed kinase in Drosophila but not in vertebrate [17] , [18] , [19] , [22] . Within the Drosophila Smo C-tail, several phosphorylation clusters are regulated by the PKA/CK1 kinases, leading to a sequential phosphorylation of Smo and resulting in a gradual activation of Hh signalling [17] , [18] , [19] , [22] , [23] , [24] , [25] , [26] . Interestingly, PKA has a dual and opposite role in the Hh pathway. In the HSC, in the absence of Hh, PKA phosphorylates Ci155 (or Gli2/3) at several Ser/Thr residues, thereby priming it for further phosphorylation [27] , [28] ; this induces partial proteolysis and formation of Ci-Rep ( Fig. 1b ) and Gli2/3-R. In contrast, in Drosophila the progressive induction of Hh pathway leads to the accumulation and phosphorylation of Smo by PKA [17] , [18] , [19] in the HSC, blocking the formation of Ci-Rep and leading to the accumulation and activation of Ci155 ( Fig. 1b ). Thus, PKA acts as both inhibitory and activating factor, but it is unclear how these different activities are regulated by the Hh pathway. Here we provide evidences that the PKA is constitutively associated to the Cos2/Fu complex, in the presence or absence of Hh signalling, and that the Cos2/Fu complex is necessary for both PKA-dependent Ci and Smo phosphorylation. We also show that Hh activation triggers changes within the HSC in the Ci/Smo stoichiometry, resulting in a switch of substrate recognition by PKA, from Ci to Smo. These data clarify another important step on the hierarchy of the intracellular events that are characterizing the Hh pathway transduction. Earlier work had demonstrated that altering the serine at position 687 (PKA phospho site Fig. 1a ) can nearly completely abolish Smo activation, revealing the importance of the phosphorylation at this position in the hierarchy of Smo phospho sites in the C-tail [17] , [18] , [19] . To enable the monitoring of Smo phosphorylation resulting from Hh signalling, we raised an antibody (referred to as p-Smo) against Smo phospho residues 687 and 690 (PKA and CK1 phospho sites, respectively, Fig. 1a ); this antibody showed both in vitro and in vivo specificity for phosphorylated Smo ( Fig. 1b–e ). In Hh-activated cultured cells, phosphorylation was observed on the endogenous form of Smo ( Fig. 1b ) and on a Smo-GFP wild-type (WT) protein, but not on the Smo-GFP AAA variant (in which the PKA and CK1 phospho sites are replaced with alanine [17] ( Fig. 1c ). In vivo , the distribution of p-Smo was similar to that of the Smo protein ( Fig. 1d ). In the anterior cells, the stabilization and phosphorylation of Smo has been shown to promote Ci155 accumulation ( Fig. 1d ), in an overlapping gradient clearly observed in the absence of GPRK2 (ref. 23 ), a kinase which regulates Smo level ( Fig. 1f ). Expression of SmoWT in the P compartment, where Hh signalling is constitutively activated, increased p-Smo detection ( Fig. 1e ). In contrast, expressing the SmoWT transgene in the anterior-most cells of the A compartment, where Hh signalling is absent, increased the Smo protein level without concomitantly increasing the level of phosphorylated Smo ( Fig. 1e ). Further, the levels of both Smo protein and Smo phosphorylation were increased in anterior ptc mutant clones, in which Hh signalling is strongly activated [5] ( Fig. 2a ). Finally, no p-Smo signal was detected in cells expressing double-stranded RNA (dsRNA) against Smo ( Fig. 2b ) or expressing Smo-GFP AAA ( Fig. 2c ). 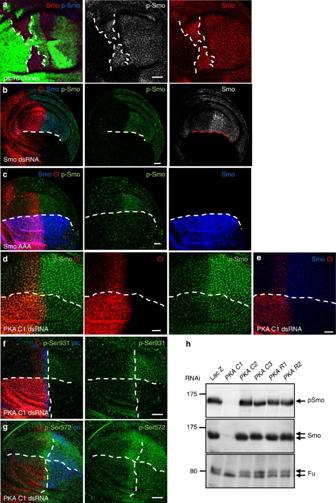Figure 2: The PKA subunit C1 is necessary for Smo phosphorylation and stabilization. (a) Wing disc expressingptcloss-of-function clones (marked by the absence of GFP) was stained for p-Smo (blue,aand grey,a) and Smo (red,a). (b,c) Wing discs expressing UAS-Smo dsRNA against Smo (b) or UAS-Smo AAA (c) driven by ap-Gal4 were stained for Ci (red,b,c), p-Smo (green,b,c) and Smo (blue,b,cand grey,b). (d–g) Wing discs expressing UAS PKA-C1 dsRNA with ap-Gal4 were stained with Ci (red,d–f,g), Smo (blue,e), Cos2 pSer931 (green,f), Cos2 p572 (green,g),ptc(blue,f) anden(blue,g). (h) S2R+ cells were transfected with dsRNA against the different PKA subunits and cell lysates were analysed by western blotting. Scale bars, 20 μm. Figure 2: The PKA subunit C1 is necessary for Smo phosphorylation and stabilization. ( a ) Wing disc expressing ptc loss-of-function clones (marked by the absence of GFP) was stained for p-Smo (blue, a and grey, a ) and Smo (red, a ). ( b , c ) Wing discs expressing UAS-Smo dsRNA against Smo ( b ) or UAS-Smo AAA ( c ) driven by ap-Gal4 were stained for Ci (red, b , c ), p-Smo (green, b , c ) and Smo (blue, b , c and grey, b ). ( d – g ) Wing discs expressing UAS PKA-C1 dsRNA with ap-Gal4 were stained with Ci (red, d – f , g ), Smo (blue, e ), Cos2 pSer931 (green, f ), Cos2 p572 (green, g ), ptc (blue, f ) and en (blue, g ). ( h ) S2R+ cells were transfected with dsRNA against the different PKA subunits and cell lysates were analysed by western blotting. Scale bars, 20 μm. Full size image To investigate which of the three catalytic subunits of Drosophila PKA regulates Smo phosphorylation, dsRNA against each of the subunits was expressed in cultured cells or in wing discs. A strong decrease of p-Smo was observed when the catalytic subunit 1 (PKA-C1) was depleted with dsRNA ( Fig. 2d-e,h ). As previously described, the lack of PKA-C1-dependent phosphorylation of Smo reduced Smo level [18] . No effect was observed with dsRNA against either of the other catalytic or regulatory subunits ( Fig. 2h ). The expression of dsRNA against PKA-C1 also lowered the levels of phosphorylated Fu and Cos2 ( Fig. 2f–h ), presumably resulting from the reduction in Hh signalling downstream of Smo [17] , [18] , [19] , [20] , [21] , [29] . Although Smo is known to be phosphorylated by PKA, the nature of how the association between these two proteins is regulated remains elusive. Two other proteins present in the HSC, Fu and Cos2, are constitutively associated and Cos2 stabilizes Fu level [7] . To examine the role of the Cos2/Fu complex in PKA-dependent Smo phosphorylation, we expressed dsRNA against either Cos2 or Fu in the dorsal compartment of the wing disc. To avoid feedback regulatory loops, we focused our attention on the P compartment, as Smo stabilization is constitutive in this compartment independently of Ptc regulation and does not trigger a transcriptional response because of the lack of Ci expression. As with PKA-C1 ( Fig. 2d,e ), decreasing the level of either Cos2 or Fu lowered the levels of p-Smo both in vivo and in vitro ( Fig. 3a,b,d ). On contrary, overexpressing both Cos2 and Fu or a dead variant of Fu kinase (Fu-HA-KD) strongly increased the levels of both Smo and p-Smo in both the wing imaginal disc ( Fig. 3c ) and in cultured cells ( Fig. 3e ). These results suggested that the phosphorylation of Smo at the PKA site requires both Cos2 and Fu. To confirm the proximity between PKA and Smo within the Cos2/Fu complex in vivo , we used a transgenic construct (Kinco) expressing a Cos2 chimera protein in which the Cos2 motor domain was replaced by the kinesin motor domain of a classical kinesin [11] . In the wing imaginal disc, it has been shown that expression of Kinco, in which binding sites for Smo, Fu and Ci are conserved, induced the relocalization of the PKA and Ci proteins at the basal membrane of polarized cells ( Fig. 4c,e ) [11] . Interestingly, expression of Kinco also induced a relocalization of Smo and pSmo with PKA and Ci at the basal side of the cells ( Fig. 4a,d,e ). Moreover, a strong decrease of p-Smo in the Kinco complex was observed when PKA-C1 was depleted with dsRNA ( Fig. 4b, f-g ). 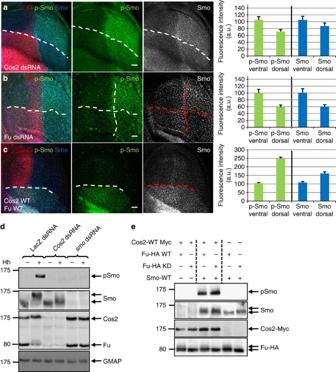Figure 3: The Cos2/Fu complex controls the PKA-dependent phosphorylation of Smo. (a–c) Wing discs expressing dsRNA against Cos2 (a), Fu (b) or Cos2-WT and Fu-WT (c) using ap-Gal4 were stained for Ci (red,a–c), p-Smo (green,a–c) and Smo (blue,a–cand grey,a–c). The A/P and D/V borders are indicated by dashed lines. Related quantification graphs (n=5, mean ±s.d) of stainings in the posterior compartment are shown on the right.bNote that in the anterior-dorsal cells depleted forfu, Smo is stabilized, which is likely to be due to the lack of the Fu-dependent Ptc expression, but not phosphorylated. (d,e) S2R+ and Hh-expressing S2R+ cells were transfected with indicated dsRNA (d) or constructs (e), and lysates were analysed by western blotting for the presence of indicated proteins. Note that decreasing Cos2 level by RNAi decreased Fu level as previously shown7. Scale bars, 20 μm. Figure 3: The Cos2/Fu complex controls the PKA-dependent phosphorylation of Smo. ( a – c ) Wing discs expressing dsRNA against Cos2 ( a ), Fu ( b ) or Cos2-WT and Fu-WT ( c ) using ap-Gal4 were stained for Ci (red, a–c ), p-Smo (green, a – c ) and Smo (blue, a – c and grey, a – c ). The A/P and D/V borders are indicated by dashed lines. Related quantification graphs ( n =5, mean ±s.d) of stainings in the posterior compartment are shown on the right. b Note that in the anterior-dorsal cells depleted for fu , Smo is stabilized, which is likely to be due to the lack of the Fu-dependent Ptc expression, but not phosphorylated. ( d , e ) S2R+ and Hh-expressing S2R+ cells were transfected with indicated dsRNA ( d ) or constructs ( e ), and lysates were analysed by western blotting for the presence of indicated proteins. Note that decreasing Cos2 level by RNAi decreased Fu level as previously shown [7] . Scale bars, 20 μm. 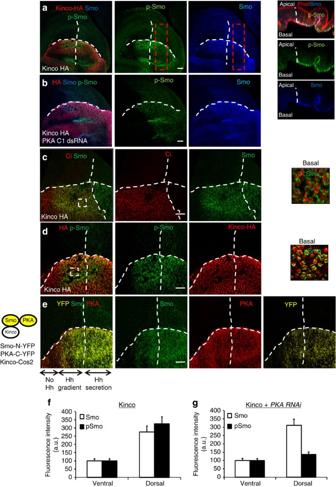Figure 4: Smo, PKA and Ci proteins colocalize with Kinco-Cos2. (a–d) Wing discs expressing HA-Kinco in the presence of dsRNA against PKA-C1 (b) or not (a,c,d), driven with ap-Gal4, was immunostained with HA (red,a,b,d), pSmo (green,a,b,d), Smo (blue,a,band green,c) and Ci (red,c). (a) On the right of the panel, a large magnification Z view of the disca(red square) is shown ina (phalloïdin, in red). pSmo and Smo are enriched at the a basal side of the wing disc epithelium. (c,d) On the right, magnifications of cells expressing Kinco-Cos2; (White square) note the relocalization of Ci (red) with Smo (green) (c) and Kinco (red) with pSmo (d) at the basal side of wing discs. (e) Wing discs expressing PKA-C-YFP and Smo-N-YFP in the presence of Kinco were stained for Smo (green,e) and PKA (red,e). YFP BiFC signals were detected in yellow ine. Reconstitution of YFP activity between PKA and Smo reveals that Smo interacts gradually with PKA in the Fu/Cos2 complex of the anterior cells. (f,g) Related quantification graph of stainings shown inaandb(n=3, mean ±s.d). Scale bars, 20 μm. Full size image Figure 4: Smo, PKA and Ci proteins colocalize with Kinco-Cos2. ( a – d ) Wing discs expressing HA-Kinco in the presence of dsRNA against PKA-C1 ( b ) or not ( a , c , d ), driven with ap-Gal4, was immunostained with HA (red, a , b , d ), pSmo (green, a , b , d ), Smo (blue, a , b and green, c ) and Ci (red, c ). ( a ) On the right of the panel, a large magnification Z view of the disc a (red square) is shown in a ( phalloïdin, in red). pSmo and Smo are enriched at the a basal side of the wing disc epithelium. ( c , d ) On the right, magnifications of cells expressing Kinco-Cos2; (White square) note the relocalization of Ci (red) with Smo (green) ( c ) and Kinco (red) with pSmo ( d ) at the basal side of wing discs. ( e ) Wing discs expressing PKA-C-YFP and Smo-N-YFP in the presence of Kinco were stained for Smo (green, e ) and PKA (red, e ). YFP BiFC signals were detected in yellow in e . Reconstitution of YFP activity between PKA and Smo reveals that Smo interacts gradually with PKA in the Fu/Cos2 complex of the anterior cells. ( f , g ) Related quantification graph of stainings shown in a and b ( n =3, mean ±s.d). Scale bars, 20 μm. Full size image To further investigate the role of Cos2/Fu in the regulation of PKA, we next asked whether endogenous PKA is present within Cos2/Fu complexes obtained by immunoprecipitating Cos2 from S2R+ cells that had been activated or not by Hh ( Figs 1b and 5a,b ). As previously reported, endogenous PKA was present within the Cos2/Fu complex in the absence of Hh ( Fig. 5a,b , lanes 3). Surprisingly, however, we also observed PKA within the complex in cells activated by Hh, in contrast to previous work [11] ( Figs 1b and 5a , lane 4). PKA was also associated with Smo and with phosphorylated Cos2 on Hh signalling activation ( Fig. 5a,b , lane 6 and lane 2, respectively). 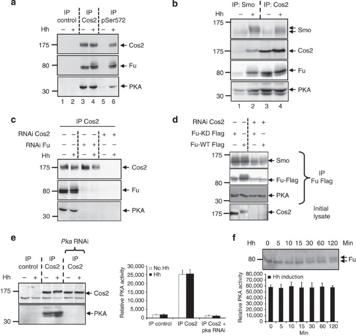Figure 5: PKA is constitutively active within the Cos2/Fu complex. (a,b) Extracts from cl8 and Hh-expressing cl8 cells were subjected to immunoprecipitation with Armadillo (control), Cos2, Cos2 p-Ser572 and Smo antibodies, and the immunoprecipitates were analysed by western blotting for the presence of Smo, Cos2, Fu and PKA. (c) S2 R+ and S2 R+ expressing Hh were transfected or not with Fu dsRNA or Cos2 dsRNA. Lysates were immunoprecipitated with an anti-Cos2 antibody and analysed for the presence of PKA. (d) S2R+ cells expressing Hh were transfected with the indicated constructs and cell lysates were subjected to immunoprecipitation with Cos2 (c) or Flag (d) antibody. Immunoprecipitates were analysed for the presence of the indicated proteins. (e) S2 R+ and S2 R+ expressing Hh were transfected or not with PKA-C1 dsRNA and lysates were immunoprecipitated with an anti-Cos2 antibody. Immunoprecipitates were analysed by western blotting for the presence of the Cos2/PKA complex, and PKA activity in the protein complex was measured by adding a peptide substrate in the presence of ATP. The level of peptide phosphorylation was measured by a luminescent PKA assay. Quantification of PKA activity is presented in the graph on the right (n=3, mean ±s.d). (f) S2 R+ cells expressing Hh under the control of the metallothionein promoter were induced for the indicated times (in minutes) with CuSO4. Similar to that ine, Cos2 immunoprecipitates were analysed by western blotting and PKA activity (graph). Figure 5: PKA is constitutively active within the Cos2/Fu complex. ( a , b ) Extracts from cl8 and Hh-expressing cl8 cells were subjected to immunoprecipitation with Armadillo (control), Cos2, Cos2 p-Ser572 and Smo antibodies, and the immunoprecipitates were analysed by western blotting for the presence of Smo, Cos2, Fu and PKA. ( c ) S2 R+ and S2 R+ expressing Hh were transfected or not with Fu dsRNA or Cos2 dsRNA. Lysates were immunoprecipitated with an anti-Cos2 antibody and analysed for the presence of PKA. ( d ) S2R+ cells expressing Hh were transfected with the indicated constructs and cell lysates were subjected to immunoprecipitation with Cos2 ( c ) or Flag ( d ) antibody. Immunoprecipitates were analysed for the presence of the indicated proteins. ( e ) S2 R+ and S2 R+ expressing Hh were transfected or not with PKA-C1 dsRNA and lysates were immunoprecipitated with an anti-Cos2 antibody. Immunoprecipitates were analysed by western blotting for the presence of the Cos2/PKA complex, and PKA activity in the protein complex was measured by adding a peptide substrate in the presence of ATP. The level of peptide phosphorylation was measured by a luminescent PKA assay. Quantification of PKA activity is presented in the graph on the right ( n =3, mean ±s.d). ( f ) S2 R+ cells expressing Hh under the control of the metallothionein promoter were induced for the indicated times (in minutes) with CuSO4. Similar to that in e , Cos2 immunoprecipitates were analysed by western blotting and PKA activity (graph). Full size image To determine which member of the Cos2/Fu complex PKA interacts with, we treated S2R+ cells with dsRNA against either Fu or Cos2 and examined the level of endogenous PKA in Cos2 or Fu immunoprecipitates, respectively. As shown in Fig. 5c , PKA was no longer associated with Cos2 in the absence of Fu. In contrast, both Fu-WT and a kinase-dead version of Fu (Fu-KD) still co-precipitated with PKA in the absence of Cos2 ( Fig. 5d ), strongly suggesting that it is Fu, and not Cos2, that acts to bring PKA into proximity to Smo, allowing Smo phosphorylation. Taken together, these results revealed a constitutive association of PKA with the Cos2/Fu complex that is independent of Hh signalling. Having observed that PKA constitutively associates with the Cos2/Fu complex independently of Hh signalling, we next wanted to determine whether the PKA activity within the complex was also independent of Hh. To this end, Cos2/Fu-associated PKA was immunoprecipitated from Drosophila cell extracts and a PKA peptide substrate was added in the presence of ATP. In this assay, local PKA associated with the HSC had the same level of activity whatever the levels of Hh induction ( Fig. 5e,f ), suggesting that the PKA present within the Cos2/Fu complex is active and that this activity is not regulated by Hh. As in absence of Hh, Ci is proteolytically cleaved subsequent to phosphorylation by PKA in a reaction that depends on the Cos2/Fu complex [11] , we investigated whether Cos2/Fu regulates PKA-dependent Ci phosphorylation similar to how it regulates Smo phosphorylation. We first transfected tagged constructs of PKA, Ci, Cos2 and Fu into S2R+ cells, and precipitated PKA with anti-HA antibodies. Although the full-length protein or part of the C-terminal domain of Fu (aa 303 to 669) were always found associated with PKA, Cos2 and Ci were only pulled down with PKA when the end of the C-terminal domain of Fu (aa 670 to 802) involved in Cos2 interaction [13] was also present ( Supplementary Fig. 1a ). Next, we expressed dsRNA against Fu, Cos2 or PKA-C1 in the dorsal compartment of the wing imaginal disc. In WT disc, the unprocessed form of Ci (Ci-155) can be detected in Hh-receiving cells anterior to the A/P border. Beyond the limits of Hh influence, Ci-155 is cleaved and converted into a truncated protein (Ci-75) not detected by the anti-Ci155 antibody ( Fig. 6a ). In all three dsRNA conditions, Ci-155 was observed throughout the A compartment, indicating that Ci processing, and hence phosphorylation by PKA, did not occur ( Fig. 6b–d,j ). As shown previously [30] , [31] , similar stabilization of Ci-155 in the A compartment was observed in mutant clones depleted for fu ( fuZ4 ), or in a class II fu mutant animal ( fuA ) lacking the Fu C-terminal domain [32] ( Fig. 6e,f,j ). In contrast, Ci processing was unaffected in cells expressing Fu-KD or in a class I fu mutant ( fu1 ) containing an inactivating mutation in the kinase domain [31] , [32] ( Fig. 6g–i ). Protein immunoprecipitation from imaginal disc lysates showed that Fu1 protein formed an intact complex with PKA and Cos2, whereas class II Fu mutant protein [32] is associated with PKA but not with Cos2 ( Supplementary Fig. 1b ). As depletion of Fu or Cos2 strongly decreased both Ci processing and Smo phosphorylation ( Figs 3a,b and 6b,c ), it seemed likely to be that the integrity of the Cos2/Fu complex, but not necessarily the Fu kinase activity itself, was necessary for the PKA-dependent phosphorylation of Ci and Smo. Together, our data reveal similar mechanisms in the regulation by the Cos2/Fu complex of the PKA-mediated phosphorylation of Smo and Ci, and suggest that the presence of Fu, but not its kinase activity, is necessary to bring PKA close to its substrates which are associated with Cos2 protein. 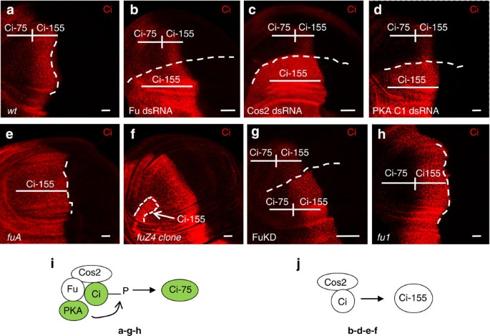Figure 6: Fu is necessary for the PKA-dependent Ci processing. (a) Wild-type wing disc was stained for Ci155 (red) using the 2A1 antibody, which recognizes C-terminal epitopes on Ci. Ci-155 can be detected in about seven rows of Hh-receiving cells anterior to the A/P border in the wing imaginal disc. In contrast, further anteriorly, beyond the limits of Hh influence, Ci-155 is cleaved and converted into Ci-75 that acts as a transcriptional repressor, which is not detected by the anti-Ci antibody. Domains of Ci-75 and Ci-155 are indicated on discs. (b–f) Wing discs expressing UAS-Fu dsRNA (b), UAS-Cos2 dsRNA (c) and UAS-PKA-C1 dsRNA (d) driven by ap-Gal4, and wing discs fromfuAmutant (e) orfuZ4mutant clones (f) were stained for Ci (red). (g,h) Wing discs expressing Fu-KD (g) orfu1mutants (h) are stained for Ci (red). (i,j) Schematic representation of different genetic backgrounds: ina,g,hintact complex, whereas inb,d,e,fFu and PKA are absent from the Cos2/Ci complex. Scale bars, 20 μm. Figure 6: Fu is necessary for the PKA-dependent Ci processing. ( a ) Wild-type wing disc was stained for Ci155 (red) using the 2A1 antibody, which recognizes C-terminal epitopes on Ci. Ci-155 can be detected in about seven rows of Hh-receiving cells anterior to the A/P border in the wing imaginal disc. In contrast, further anteriorly, beyond the limits of Hh influence, Ci-155 is cleaved and converted into Ci-75 that acts as a transcriptional repressor, which is not detected by the anti-Ci antibody. Domains of Ci-75 and Ci-155 are indicated on discs. ( b – f ) Wing discs expressing UAS-Fu dsRNA ( b ), UAS-Cos2 dsRNA ( c ) and UAS-PKA-C1 dsRNA ( d ) driven by ap-Gal4, and wing discs from fuA mutant ( e ) or fuZ4 mutant clones ( f ) were stained for Ci (red). ( g , h ) Wing discs expressing Fu-KD ( g ) or fu1 mutants ( h ) are stained for Ci (red). ( i , j ) Schematic representation of different genetic backgrounds: in a , g , h intact complex, whereas in b , d , e , f Fu and PKA are absent from the Cos2/Ci complex. Scale bars, 20 μm. Full size image We next investigated the mechanism underlying the switch that occurs in PKA targeting from Ci to Smo on increased Hh signalling. We first identified the PKA binding sites within Smo (Smo581-798aa) and Ci (Ci720-1009aa); these sites were present within specific domains located around the PKA phosphorylation sites on each protein ( Fig. 7a,c ). As the level of Smo increases on Hh activation, we wondered whether the presence of Smo in cells could somehow change the interaction of PKA with Ci. To test this possibility, we transfected constructs expressing PKA together with either full-length Smo-WT or Ci-WT into Sf9 cells ( Fig. 7b ) or Drosophila cells ( Supplementary Fig. 2a ), immunoprecipitated with anti-PKA antibodies, and measured the relative abundance of associated Smo-WT or Ci-WT. The two proteins interacted with PKA with the same effectiveness ( Fig. 7b , compare lanes 3 and 4). Interestingly, however, when we co-expressed Smo-WT and Ci-WT at similar levels, the interaction between PKA and Smo was favoured ( Fig. 7b , lane 6), whereas Smo mutant lacking the binding site of PKA did not compete with Ci-WT ( Supplementary Fig. 2b , lanes 3 and 5). To further confirm this difference, we performed a competition assay using the different Ci and Smo binding domains for PKA, in which constant amounts of Ci720-1009aa and PKA were expressed together with increasing amounts of Smo581-798aa ( Fig. 6d ). We observed that the PKA-Ci interaction gradually decreased with increasing levels of Smo ( Fig. 6d ), suggesting that Ci and Smo compete for PKA binding, and confirming that PKA has a higher affinity for Smo than for Ci. Together, these results suggest a mechanism by which Hh induces a switch in PKA targeting, from Ci to Smo, by increasing the level of Smo. 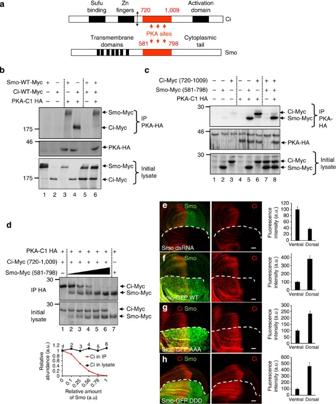Figure 7: Smo competes with Ci for PKA binding. (a) Schemes of the Ci and Smo proteins. (b) Sf9 cells were transfected with the indicated constructs. Cell lysates were subjected to immunoprecipitation with antibody against HA and were analysed for the presence of the indicated proteins. (c) S2 R+ cells were transfected with PKA-C1-HA and the domain covering the PKA-binding sites of Ci-Myc (aa720-1009) and Smo-Myc (aa581-798). Ind, PKA-HA was co-expressed with increasing amounts of Smo-Myc (aa581-798) and a fixed amount of Ci-Myc (aa720-1009). Inb,c,d, PKA-HA immunoprecipitates and initial lysates were analysed for the presence of the indicated proteins. (d) Relative quantification of Smo and Ci present in the initial lysate and the PKA immunoprecipitates. Note that Smo competes with Ci for PKA (inblane 6 andclane 8). (e–h) Wing discs expressing UAS-Smo-dsRNA (e), UAS-Smo-WT (f), UAS-Smo-AAA (g) and UAS-Smo-DDD (h) using ap-Gal4 were stained for Ci155 (red,e–h) and Smo (green,e–h). Related quantification graphs of Ci staining in the anterior compartment are shown on the right (n=3, ±s.d.). Scale bars, 20 μm. Figure 7: Smo competes with Ci for PKA binding. ( a ) Schemes of the Ci and Smo proteins. ( b ) Sf9 cells were transfected with the indicated constructs. Cell lysates were subjected to immunoprecipitation with antibody against HA and were analysed for the presence of the indicated proteins. ( c ) S2 R+ cells were transfected with PKA-C1-HA and the domain covering the PKA-binding sites of Ci-Myc (aa720-1009) and Smo-Myc (aa581-798). In d , PKA-HA was co-expressed with increasing amounts of Smo-Myc (aa581-798) and a fixed amount of Ci-Myc (aa720-1009). In b , c , d , PKA-HA immunoprecipitates and initial lysates were analysed for the presence of the indicated proteins. ( d ) Relative quantification of Smo and Ci present in the initial lysate and the PKA immunoprecipitates. Note that Smo competes with Ci for PKA (in b lane 6 and c lane 8). ( e – h ) Wing discs expressing UAS-Smo-dsRNA ( e ), UAS-Smo-WT ( f ), UAS-Smo-AAA ( g ) and UAS-Smo-DDD ( h ) using ap-Gal4 were stained for Ci155 (red, e – h ) and Smo (green, e – h ). Related quantification graphs of Ci staining in the anterior compartment are shown on the right ( n =3, ±s.d.). Scale bars, 20 μm. Full size image If this switch depends solely on the level of Smo that is capable of binding to PKA, then a similar switch should be observed with different variants of Smo, independently of their activity. To address this possibility, we expressed in Drosophila wing imaginal discs either WT (Smo-WT), inactive (Smo-AAA) [17] or constitutively active (Smo-DDD, with glutamic acid substitutions of PKA and CK1 phospho sites [17] ) forms of Smo. Expressing Smo dsRNA in the dorsal compartment of the wing disc enhanced Ci cleavage and led to an absence of Ci-155 in this domain ( Fig. 7e ). This result suggested that Ci is constitutively phosphorylated by PKA in the absence of Smo. Conversely, the expression of Smo-WT, Smo-AAA or Smo-DDD throughout the dorsal domain ( Fig. 7f–h ) or in anterior clones of cells ( Supplementary Fig. 3a–c ) led to an accumulation of Ci-155 and thus blocked the PKA-dependent cleavage of Ci. Analysis of phospho-Cos2 and Ptc level, two positive read out downstream of Smo in the Hh pathway, showed that accumulation of Ci155 depends on Smo expression but not on Smo activity ( Supplementary Fig. 3d–g ). To examine this phenomenon in vitro , we analysed the effects of Smo on PKA-dependent Ci cleavage in S2 R+ cells. After Cos2 immunoprecipitation, we examined the effects of the Smo variants on PKA-dependent Ci phosphorylation within the PKA/Smo/Fu/Cos2 complex ( Fig. 8a ). To better visualize the phosphorylation-dependent electrophoretic shift of Ci, transfected cultured cells were treated with the proteasome inhibitor MG132, which blocks the partial proteolysis of phosphorylated Ci [33] . 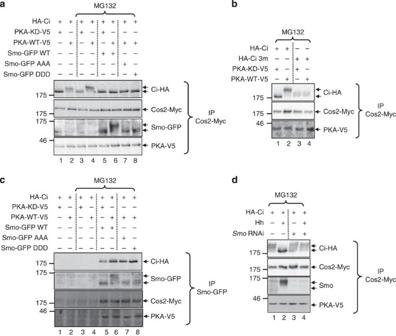Figure 8: Smo blocks the PKA/Ci processing within Cos2/Fu complex. (a–d) S2 R+ cells expressing or not Hh were transfected with the indicated constructs. In all conditions, the Cos2-Myc and Fu constructs were also transfected. Ind, cells were transfected in presence or not of dsRNA againt Smo. Cells were treated with 50 μM of MG132, and lysates were subjected to immunoprecipitation with antibodies to Cos2-Myc (a,b,d) or to Smo-GFP (c). Immunoprecipitates were analysed for the presence of the indicated proteins. Note that a Fu-KD variant was used to avoid any potential influence of Fu kinase activity in this assay, specifically to avoid dissociation of Ci from the complex. Figure 8: Smo blocks the PKA/Ci processing within Cos2/Fu complex. ( a – d ) S2 R+ cells expressing or not Hh were transfected with the indicated constructs. In all conditions, the Cos2-Myc and Fu constructs were also transfected. In d , cells were transfected in presence or not of dsRNA againt Smo. Cells were treated with 50 μM of MG132, and lysates were subjected to immunoprecipitation with antibodies to Cos2-Myc ( a , b , d ) or to Smo-GFP ( c ). Immunoprecipitates were analysed for the presence of the indicated proteins. Note that a Fu-KD variant was used to avoid any potential influence of Fu kinase activity in this assay, specifically to avoid dissociation of Ci from the complex. Full size image Immunoprecipitation of Cos2 confirmed the formation of a Cos2/Fu/PKA/Ci complex, in which most of the Ci-155 was phosphorylated by PKA ( Fig. 8a ). Phosphorylation of Ci was promoted by the expression of PKA-WT ( Fig. 8a , lane 4), but abolished in presence of PKA-KD ( Fig. 8a , lane 3). This regulation is not observed with a variant of Ci (Ci-3m) lacking three potential PKA phosphorylation sites ( Fig. 8b ), confirming the PKA-dependent regulation of Ci phosphorylation. In contrast, the presence of Smo-WT in the complex strongly reduced the level of Ci phosphorylation, while Smo was itself phosphorylated ( Fig. 8a , compare lanes 4 and 6). To confirm that this process was carried out within the same complex, Smo was immunoprecipitated and the presence of Ci was analysed in the immunoprecipitates ( Fig. 8c ). As Ci does not interact directly with Smo, presence of Ci was due to its association with the Fu/Cos2 proteins. In spite of its presence with PKA in the Smo/Fu/Cos2 complex, Ci was not phosphorylated by PKA ( Fig. 8c , lanes 5 and 6). Interestingly, the expression of either Smo-AAA or Smo-DDD similarly inhibited Ci phosphorylation within the complex ( Fig. 8a,c , lanes 7 and 8). Moreover, PKA-dependent phosphorylation of Ci within the complex was restored on depletion of endogenous Smo ( Fig. 8d compare lanes 2 and 4), confirming that the presence of Smo within the HSC blocks the phosphorylation of Ci by PKA. Together, these data suggest that Hh induces a switch in the PKA substrate, from Ci to Smo, by increasing the level of Smo within the signalosome complex. This increase in Smo would cause PKA to change its association from Ci to Smo within the complex, leading to the phosphorylation of Smo instead of Ci. To further address this possibility, we next examined the interactions between PKA and Ci and Smo within the Cos2/Fu complex in living cells, using the multicolour BiFC technique [34] . Two non-fluorescent fragments of a split yellow fluorescent protein (YFP) were fused separately to Ci and PKA, and additional tags were inserted to enable the proteins to be followed by immunohistochemistry ( Fig. 9 ). Using this system, an interaction between PKA-C-YFP with Ci-N-YFP would bring the two non-fluorescent fragments into close proximity, thereby reconstituting an intact fluorescent YFP. For these experiments, we used the Ci-3m variant, which can interact with PKA without being partially degraded [27] . We analysed the subcellular localizations of Ci-3m and PKA in S2R+ cells, and analysed the effect of Hh on their interactions by measuring YFP activity, in the presence or the absence of Cos2, Fu and Smo constructs. In the presence of exogenous Cos2/Fu complex, Ci-N-YFP and PKA-C-YFP colocalized within punctate structures ( Fig. 9a ) that were positive for both Cos2 and Fu ( Supplementary Fig. 4b ), and a strong YFP signal was detected. Depletion of endogenous Cos2 ( Supplementary Fig. 4f ) or absence of exogenous Fu/Cos2 ( Supplementary Fig. 4a ) did not give a significant YFP signal. These observations confirmed the existence of a close interaction between Ci and PKA within the Cos2/Fu complex. Expression of either Ci3m-N-YFP or PKA-C-YFP alone, or the co-transfection of split cytoplasmic N- and C-YFP fragments, or the co-transfection with a construct expressing a control Ci3m-N-YFP construct deleted for the PKA-binding site ( Supplementary Fig. 4e,i,j ) did not induce YFP reconstitution at a significant level in the presence of the Cos2/Fu complex. 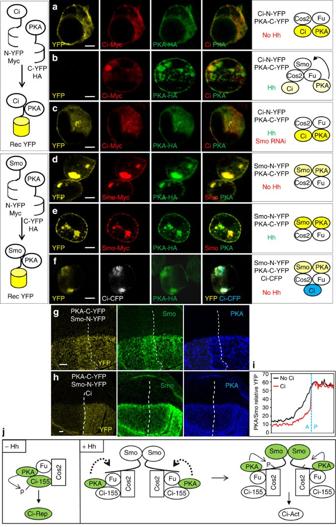Figure 9: Association-switch of PKA from Ci towards Smo. (a–f) S2 R+ cells transfected with Ci-N-YFP-Myc or Smo-N-YFP-Myc and PKA-C-YFP-HA in the presence of Cos2/Fu and Ci-CFP (f). Ci used in BiFC experiment is a Ci variant, Ci3m, in which the PKA sites were substituted for alanine. Schematic representations of reconstitution of YFP activity are indicated on the left, while the conditions and structure of signalosome complex are indicated on the right of each panel. Transfected cells were stained for Myc (red ina–e) and HA (green ina–f). YFP signals were detected in yellow fora–f. Ci-CFP is visualized in grey infand in blue inf. Quantifications of different transfection conditions are presented inSupplementary Fig. 4g and 5h. (g,h) Wing imaginal discs co-expressing in the dorsal compartment (with the use of the apterous-Gal4 driver) UAS-Smo-N-YFP and UAS-PKA-C-YFP in the presence (h) or not (g) of Ci-CFP were stained for Smo (green,g,h) and PKA (blue,g,h). YFP signals were detected in yellow forgandh. Quantifications of YFP reconstitution in wing imaginal discs are shown ini. (j) Scheme representing the association switch of PKA from Ci to Smo within the Cos2/Fu complex. In the absence of Hh, degradation of Smo and PKA/Ci interactions facilitate the PKA-dependent phosphorylation and processing of Ci. On induction, Hh promotes the stabilization of Smo, which associates with the Fu/Cos2 complex and displaces PKA from Ci, leading to Smo phosphorylation and activation. Scale bars, 5 μm (cells) or 20 μm (discs). Figure 9: Association-switch of PKA from Ci towards Smo. ( a – f ) S2 R+ cells transfected with Ci-N-YFP-Myc or Smo-N-YFP-Myc and PKA-C-YFP-HA in the presence of Cos2/Fu and Ci-CFP ( f ). Ci used in BiFC experiment is a Ci variant, Ci3m, in which the PKA sites were substituted for alanine. Schematic representations of reconstitution of YFP activity are indicated on the left, while the conditions and structure of signalosome complex are indicated on the right of each panel. Transfected cells were stained for Myc (red in a – e ) and HA (green in a – f ). YFP signals were detected in yellow for a – f . Ci-CFP is visualized in grey in f and in blue in f . Quantifications of different transfection conditions are presented in Supplementary Fig. 4g and 5h . ( g , h ) Wing imaginal discs co-expressing in the dorsal compartment (with the use of the apterous-Gal4 driver) UAS-Smo-N-YFP and UAS-PKA-C-YFP in the presence ( h ) or not ( g ) of Ci-CFP were stained for Smo (green, g , h ) and PKA (blue, g , h ). YFP signals were detected in yellow for g and h . Quantifications of YFP reconstitution in wing imaginal discs are shown in i . ( j ) Scheme representing the association switch of PKA from Ci to Smo within the Cos2/Fu complex. In the absence of Hh, degradation of Smo and PKA/Ci interactions facilitate the PKA-dependent phosphorylation and processing of Ci. On induction, Hh promotes the stabilization of Smo, which associates with the Fu/Cos2 complex and displaces PKA from Ci, leading to Smo phosphorylation and activation. Scale bars, 5 μm (cells) or 20 μm (discs). Full size image We examined the impact of Hh signalling on the association between PKA and Ci. Induction by Hh or expression of Smo-CFP (Smo fused to cyan fluorescent protein) induced the dissociation of PKA from Ci, as evidenced by lower level of YFP reconstitution ( Fig. 9b and Supplementary Fig. 4c,d,g,h ). It should be noted that even though there was a lack of YFP reconstitution between Ci-N-YFP and PKA-C-YFP, Smo-CFP presented multiple points of co-localization with Ci and PKA at the plasma membrane as well as in the cytoplasm ( Supplementary Fig. 4c,d ). Hence, even though PKA and Ci are both present within the HSC with Cos2, Fu and Smo, the presence of Smo in this complex prevents PKA from associating closely with Ci. To confirm this, we could show that depletion of Smo in cells activated by Hh restored the PKA/Ci interaction ( Fig. 9c and Supplementary Fig. 4g ). Altogether, the physiological increase of Smo level, observed in cells induced by Hh, inhibits PKA and Ci interaction in the HSC, and this effect is reversed on depletion of endogenous Smo. To further test the hypothesis of a shift in the association of PKA from Ci to Smo within the HSC, we also analysed the interaction between Smo-N-YFP and PKA-C-YFP by YFP complementation. When expressed separately, neither Smo-N-YFP nor PKA-C-YFP generated a YFP signal, and staining of Smo and PKA revealed a cytoplasmic localization for each of the proteins ( Supplementary Fig. 5a,b ). Conversely, when Smo-N-YFP and PKA-C-YFP were co-expressed, a YFP signal was reconstituted, both at the plasma membrane and in punctate cytoplasmic structures ( Fig. 9d and Supplementary Fig. 5c ). The YFP signal generated by the interaction between Smo-N-YFP and PKA-C-YFP strongly increased on Hh induction ( Fig. 9e and Supplementary Fig. 5d ). Depletion of endogenous Cos2 ( Supplementary Fig. 5e,f,i ), or co-transfection with a construct expressing Smo-N-YFP deleted for the PKA-binding site ( Supplementary Fig. 5g,j,k ), strongly reduced Smo and PKA interaction and YFP reconstitution. Finally, to determine whether the presence of Ci in the protein complex could influence the PKA–Smo interaction, a Ci-CFP (Ci fused to cyan fluorescent protein) construct was transfected together with Smo-N-YFP and PKA-C-YFP in the presence of the Cos2/Fu complex. Only a small decrease in the YFP signal was observed ( Fig. 9f and Supplementary Fig. 5h ), suggesting that in condition in which Ci and Smo are expressed at comparable level, Ci does not substantially compete with Smo for binding to PKA despite being present in the same complex as the two other proteins. To confirm our model, we analysed by BiFC the interaction between PKA and Smo in the wing imaginal discs. As expected, the co-expression of Smo-N-YFP and PKA-C-YFP in posterior cells, showed a Smo/PKA association at a constant level, visible with the constant BiFC signal ( Fig. 9g and graph in Fig. 9i ). Importantly, the expression of the two proteins in the anterior compartment led to a gradient of BiFC signal, suggesting a gradient of PKA/Smo interactions in anterior cells, which receive the Hh signal. Morever, expression of Kinco-Cos2 confirmed that Smo associates with PKA gradually in the Cos2/Fu complex of the anterior cells ( Fig. 4e ). Expression of either Smo-N-YFP or PKA-C-YFP alone did not induce YFP reconstitution at a significant level ( Supplementary Fig. 6 ). Unfortunately, our attempt to visualize an interaction between PKA-C-YFP and Ci-N-YFP in vivo did not succeed, leading to the absence of a significant visible BiFC signal. To circumvent this effect, we analysed the consequence of increasing the level of Ci on the PKA/Smo interaction and found that increased level of Ci changed significantly the slope of the PKA/Smo interaction gradient in the anterior compartment ( Fig. 9h-i ). This data suggest that Ci is able to interfere with the PKA/Smo interaction, and that Ci and Smo compete for PKA association in this in vivo conditions. Despite the many years that have passed since the initial discovery of PKA in the regulation of Hh-dependent patterning activity, the precise mechanism of PKA regulation within the Hh pathway has remained unclear. We show here that Smo has the potential to block productive interaction between Ci and PKA in the HSC. Our data suggest that Hh blocks Ci processing without dissociation of the Cos2/Fu/ PKA/Ci complex. Once activated, Ci dissociates from the HSC for nuclear translocation [7] , [8] , [9] , [10] , [11] , [12] , [13] , [14] , [15] , [16] , [17] , [18] , [19] , [20] , [21] , [22] , [23] , [24] , [25] , [26] , [27] , [28] , [29] , [30] , [31] , [32] , [33] . In the Smo immunoprecipitation presented here ( Fig. 8 ), Ci is still present in the activated HSC, but is not phosphorylated by PKA, while Smo is. This experiment was designed in the presence of a Fu-KD version, to avoid the dissociation of Ci from the activated complex [21] . Regardless of the Smo isoforms used—WT, constitutive active, or non-active—Smo protein blocks the conversion of Ci into the repressor form in vivo and stabilize Ci at a level similar to endogenous Ci present at the A/P border ( Supplementary Fig. 3 ), suggesting that Smo protein level and not Smo activity is involved in the blockade of Ci processing. Our in vitro data suggest that the increase in Smo level induced by Hh signalling is sufficient to outcompete Ci for PKA association. For example, we show that Hh treatment provided an accurate physiological increase of Smo ( Fig. 1b ) with dissociation of the PKA/Ci interaction observed by BiFC and this effect is reversed by depletion of endogenous Smo ( Fig. 9 ). Unfortunately, we could not test accurately this model in vivo , but we do observe formation of a Ci/Cos2/PKA/phospho-Smo complex in the wing discs ( Fig. 4 ) and we could show that increased level of Ci is able to interfere with the PKA/Smo BiFC interaction and change significantly the slope of the PKA/Smo interaction gradient in the anterior compartment ( Fig. 9 ). We propose that the Hh-dependent variations in the level of Smo within the HSC trigger changes in the Ci/Smo stoichiometry, inducing a shift in substrate recognition by PKA ( Fig. 9j ). As the Ci and Smo competition for PKA binding was done in Sf9 cells in the absence of Fu and Cos2, or in large excess of Ci and Smo peptides compared with endogenous Cos2/Fu ( Fig. 7 ), we do not believe that intermediate proteins are involved in the shift of substrate recognition by PKA. It is well accepted that two types of HSC are observed, a Fu/Cos2/PKA/Ci repressor (R) complex and a Fu/Cos2/PKA/Ci/Smo activator (A) complex, but the transition between the HSC R to A has been often eluded. It has been proposed that PKA dissociates and traffic from HSC R to A [11] . Our data demonstrate this is not the case. In the absence of Hh imput, the absence of Smo in the HSC R allows interaction of PKA with Ci, leading to the formation of Ci-Rep. We propose that the activation of the Hh pathway promotes the increase level of Smo and its association within the HSC R, abolishing the PKA/Ci interaction and thus formation of Ci-Rep, and subsequently leading to the phosphorylation of Smo and gradually to HSC A ( Fig. 9j ). In addition to this regulation, it is possible that PKA is further regulated through activation of a G protein associated to the Smo/Fu/Cos2 complex [35] . Indeed, it has been proposed that PKA induces different levels of Smo activation by promoting different cluster of phosphorylation sites [18] . It is thus possible that the combined action of G protein and PKA regulates the degree of Smo activation. Despite the differences in primary sequence between Drosophila and vertebrate Smo, in both cases Hh induces Smo phosphorylation at multiple sites, by PKA in Drosophila and by CKIalpha in vertebrates [22] , and this phosphorylation causes Smo to adopt its active conformation and correct subcellular localization. CKIalpha also induces the phosphorylation of Gli2, triggering the formation of Gli2R [36] . It is thus likely to be that a similar switch in CKIalpha targeting occurs within the vertebrate HSC on changes in the vertebrate Smo level. During the final revision of this work, Li et al. 2014 presented an independent line of evidence for a formation of a complex between Smo and PKA that induces the activation of the Hh pathway [37] . Genetics Alleles used here were reported previously: gprk2 ko [21] , fu 1 , fuA , fu RX2 , fu Z4 and ptc 16 (refs 21 , 29 ). Clones were generated as described [7] . Transgenic flies were as follows: UAS-Smo-N-YFP, UAS-PKA-C-YFP, UAS-Kinco-HA [11] , UAS-SmoAAA [17] and UAS-SmoDDD [17] , UAS-Fu-WT [29] , UAS-Fu-KD [29] and UAS-Cos2 [29] , UAS-PKA-C1 dsRNA, UAS-Smo dsRNA, UAS-Cos2 dsRNA and UAS-Fu dsRNA (all dsRNA from the Vienna Stock Centre). The Fu-KD is an inactive version of the Fu kinase with a substitution of Gly13 by Val in the ATP-binding site. Immunostaining and miscroscopy Primary antibodies were used at the following dilutions: anti-p-Smo 1:100, anti-Smo 1:20 (20C6, DSHB), anti-Cos2 1:500 (ref. 7 ), anti-Ci155 1:10 (2A1, gift from R. Holmgren), anti-Ci-N 1:500, anti-Fu 1:200 (ref. 7 ), anti-Ptc 1:200 (5E10, DSHB), anti-En 1:500 (Invitrogen), anti-HA 1:1,000 (Roche), anti-Myc 1:500 (Santa-cruz), anti-p-CosSer572 1:400 (ref. 21 , anti-p-CosSer931 1:250 (ref. 21 ) and anti-phalloidin 1:100 (Sigma). Images were captured with a Leica DMR TCS_NT confocal microscope and analysed with Image J software. Plots were analysed as described in ref. 29 . BiFC constructs and immunostaining The pUAST-BiFC vectors were described in Gohl et al. [38] Smo, Ci3m [28] and the PKA-C1 coding region were inserted into a gateway cassette downstream of the N-YFP and C-YFP fragments, enabling the construction of the C-terminal N-YFP and C-YFP fusions. The resulting constructs — the Ci3m-Myc construct was fused to the amino terminus of YFP (N-YFP 1-173aa), PKA-HA was fused to the C terminus of YFP (C-YFP 156-239aa) and Smo-Myc was fused to the N terminus of YFP (N-YFP 1-173aa) —were then used for transfection. Transgenics expressing UAS-BiFC constructs were obtained by germline transformation using the phi31-integrase. Immunohistochemistry was performed as described in ref. 21 . For transfection experiments, an actin-Gal4 plasmid was co-transfected with pUAST vectors. For a total of 2 μg DNA, 50 ng to 0.2 μg DNA for each expression vectors with 1 μg of Act-Gal4 were used in a typical transfection using 10 μl of Lipofectamine LTX (Invitrogen). After 2 days, S2 R+ cells were fixed with 4% paraformaldehyde, permeabilized with 0.1% Triton X-100 and incubated with primary antibody for 16 h at room temperature, followed by secondary antibody staining. Primary antibodies used were anti-HA and anti-Myc. Alexa568 and Alexa647-conjugued antibodies (Invitrogen) were used as secondary antibodies. To visualize the fluorescence emissions of cells expressing different combinations of fusion proteins, we used excitation at 430 nm for CFP and 514 nm for YFP. To quantify fluorescence complementation, cells were transfected with plasmids encoding the two fusion proteins, together with a control plasmid (RFP, Red Fluorescence Protein). The relative ratio of YFP and RFP fluorescence gave a measure of the relative efficiency of the complex formation. In all BiFC quantification between 150 and 200 cells were analysed. Cell culture, transfections and complementary DNA constructs Drosophila Schneider line-2R+ (S2R+), wing imaginal disc clone 8 cells (cl8) and stably transformed cl8 cell lines were maintained as previously described [7] . For YFP-fusion constructs and various ‘tag’ constructs, PKA, Fu, Cos2, Ci and Smo were amplified by PCR and cloned by the Gateway technology (Invitrogen) in pUAST vectors. For transient gene expression, the corresponding UAS constructs were cotransfected with an actin5C-Gal4 construct in S2 R+ cells or pIE1-Gal4 in Sf9 cells. Transfection was carried out using Lipofectamine LTX or cellfectin (Invitrogen). RNA interference in cells The sequences of the dsDNAs used are described at http://www.flyrnai.org/ and dsDNAs were produced in vitro from PCR products, using T7 polymerase. DsDNA transfection into S2R+ cells was performed as previously described [17] . Antibody production A specific antibody directed against the phosphorylated Ser-687 and Ser-690 residues of Smo (p-Smo) was produced by immunizing rabbits with the synthetic phosphopeptide S R R N S* V D S* Q V S V K, coupled to keyhole limpet haemocyanin 5 (Eurogentec). The reactive antibody was purified by adsorption on a phosphopeptide affinity column, and was then purified further by substraction on a column containing the unphosphorylated Smo peptide. The resulting antibody was characterized by western blotting. Rabbit antisera against PKA-C1 were raised from amino acid 247 to 353, and antibodies were affinity purified with standard procedures. Immunoprecipitation, PKA assay and western blotting For immunoprecipitation experiments, an actin-Gal4 plasmid was co-transfected with pUAST vectors. For a total of 4 μg DNA, 0.1 to 0.5 μg DNA for each expression vectors with 2 μg of Act-Gal4 were used in a typical transfection (Lipofectamine). MG132 treatment was carried out as previously described [33] . Cultured cells were lysed 2 days after transfection in lysis buffer (20 mM Tris–HCl (pH 8), 150 mM NaCl and 1% Triton) in the presence of phosphatase inhibitors (50 mM sodium fluoride and 10 mM sodium orthovanadate) and protease inhibitors. Armadillo, Smo, Cos2 and Cos2 phosphorylated on Ser572 were immunoprecipitated as described in ref. 21 , Fu-Flag was precipitated with a mouse anti-Flag antibody (M2, Sigma) and immunocomplexes were resolved by SDS–PAGE. Western blottings were performed with antibodies against Smo, Fu, Cos2, GMAP, PKA-C1 and Flag, as described by Ranieri et al. [21] The original immunoblot data are included in Supplementary figures 7-14 . The p-Smo antibody was used at 1:500 for western blotting. After Cos2 immunoprecipitation, the enzymatic activity of PKA was measured in vitro using the Kinase-Glo Luminescent Kinase Assay (Promega) in the presence of 10 μM ATP and 50 μM of Kemptide substrate. How to cite this article: Ranieri, N. et al. Switch of PKA substrates from Cubitus interruptus to Smoothened in the Hedgehog signalosome complex. Nat. Commun. 5:5034 doi: 10.1038/ncomms6034 (2014).